Ablation of TrkB signalling in CCK neurons results in hypercortisolism and obesity Dysregulation of hypothalamic–pituitary–adrenal (HPA) axis activity leads to debilitating neuroendocrine or metabolic disorders such as Cushing’s syndrome (CS). Glucocorticoids control HPA axis activity through negative feedback to the pituitary gland and the central nervous system (CNS). However, the cellular mechanisms involved are poorly understood, particularly in the CNS. Here we show that, in mice, selective loss of TrkB signalling in cholecystokinin (CCK)-GABAergic neurons induces glucocorticoid resistance, resulting in increased corticotrophin-releasing hormone expression, chronic hypercortisolism, adrenocortical hyperplasia, glucose intolerance and mature-onset obesity, reminiscent of the human CS phenotype. Interestingly, obesity is not due to hyperphagia or decreased energy expenditure, but is associated with increased de novo lipogenesis in the liver. Our study therefore identifies CCK neurons as a novel and critical cellular component of the HPA axis, and demonstrates the requirement of TrkB for the transmission of glucocorticoid signalling. Excessive levels of glucocorticoids can lead to serious metabolic dysfunctions such as Cushing’s syndrome (CS). While endogenous CS is rare and generally results from a pituitary or adrenal tumour, exogenous CS is the more common form and is caused by long-term glucocorticoid treatment. CS resembles the metabolic syndrome, with abdominal obesity, insulin resistance and type II diabetes [1] , [2] . Glucocorticoids (cortisol in humans/primates, and corticosterone (CORT) in rodents) are steroid hormones whose levels are controlled by the hypothalamic–pituitary–adrenal (HPA) axis and a physiological negative feedback loop. Upon HPA axis activation, the neurosecretory neurons in the hypothalamic paraventricular nucleus (PVN) release corticotropin-releasing hormone (CRH) into the hypophyseal portal blood stream. CRH triggers secretion of adrenocorticotropic hormone (ACTH) from the anterior pituitary, which then stimulates the adrenal glands to release glucocorticoids into the peripheral blood stream [3] , [4] , [5] . Excess circulating glucocorticoids in turn negatively affects CRH release and ACTH secretion, so modulating further glucocorticoid release by the adrenal glands. This feedback inhibition is mediated by the glucocorticoid receptor (GR) [6] . The widespread GR expression in the brain, and its genetic manipulation, indicate the involvement of glucocorticoids in many physiological processes including synaptic plasticity, anxiety and neuroendocrine control [7] . However, the molecular mechanisms underlying the fundamental changes at the central nervous system (CNS) level are unknown. The limbic system also plays a crucial role in the regulation of HPA axis activity through a multisynaptic process integrated in the hypothalamus by local circuit neurons, surrounding and projecting to the PVN [8] . The majority of synapses in the PVN and peri-PVN are GABAergic. A significant fraction of the GABAergic synaptic inputs derive from local circuit neurons forming a ring around the PVN, consistent with the anatomical localization of the limbic afferents terminal fields [8] , [9] . Yet, the critical cell type(s) in the hypothalamus that integrate information from limbic structures into PVN activation and/or inhibition is unknown. Among the different types of GABAergic inhibitory neurons, cholecystokinin (CCK)-expressing neurons are found in several regions involved in the modulation of the HPA axis activity, in particular, the hypothalamus, but also in limbic regions [10] , [11] . The neurotrophin receptor TrkB (or NTRK2) and its ligand BDNF (brain-derived neutrotrophic factor), in addition to synaptic plasticity and learning [12] , have been shown to regulate energy balance in the adult mouse brain. In particular, Bdnf deficiency or an hypomorphic allele of Trkb induces hyperphagia and concomitant obesity [13] , [14] , [15] , [16] , [17] . In humans, a patient carrying a de novo Trkb missense mutation has shown a similar hyperphagic/obese phenotype [18] . Conversely, a Val66Met substitution in the Bdnf locus has been associated with HPA axis reactivity and an altered ability to cope with stressful situations [19] , [20] . Stress induced by acute immobilization in rodents increases Bdnf mRNA and peptide levels in the hippocampus [21] , PVN [22] and other nuclei [23] , [24] . Interestingly, mice carrying Trkb deletion in principal neurons did not show defects in HPA axis activity [25] . We report here that Trkb deletion in CCK neurons disrupts GR-mediated negative feedback at the CNS level, and results in hyperactivity of the HPA axis, with associated chronic hypercortisolism, adrenocortical hypertrophy, mature-onset obesity, glucose intolerance and hepatic steatosis; all primary features of human CS. We have therefore identified a novel mechanism of HPA axis activity regulation by the CNS uncovering CCK neurons as a critical cell type, and TrkB signalling as a critical component in feedback inhibition to the PVN. Generation of CCK-specific Trkb knockout mice To elucidate a critical neuronal subtype mediating central control of HPA axis activity mice expressing the Cre -recombinase driven by the Cck promoter ( BAC-Cck-Cre , Supplementary Fig. 1a ) were generated. The recombination pattern was determined by crossing to two different reporter lines (Z/EG and R26R-YFP [26] , [27] ). A similar expression pattern was obtained to that previously published for Cck [10] ( Fig. 1a , and Supplementary Fig. 1a ). In particular, most hypothalamic nuclei showed high YFP (yellow fluorescent protein) expression, whereas the PVN and the arcuate nucleus contained only a few YFP-expressing cells ( Supplementary Fig. 1b ). About 80% of the CCK-positive cells, and 40% of the GABA-positive cells showed Cre -mediated YFP expression ( Fig. 1b ). Conversely, Parvalbumin-positive cells did not co-localize with CCK except in rare cases ( Supplementary Fig. 1c arrowhead). Low levels of CCK expression were previously reported in some pyramidal projection neurons [28] . Equally, GFP (green fluorescent protein) expression was found in some hippocampal pyramidal cells ( Fig. 1a and Supplementary Fig. 1d ). 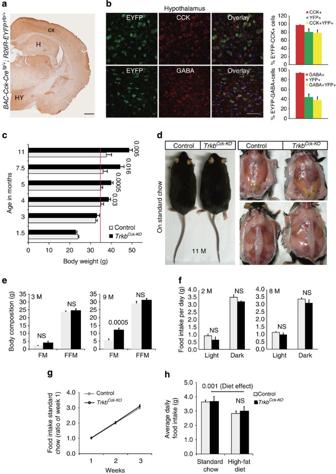Figure 1:TrkbCck-KOmice are obese but show no signs of hyperphagia. (a) Adult brain section ofBAC-Cck-Cretg/+; R26R-EYFPtg/+stained with G(Y)FP-specific antibodies (Abs).Cre-mediated EYFP expression is detected in the hypothalamus (HY), cortical layers IV and V (CX) and hippocampus (H). (b) Cellular specificity ofCre-mediated recombination was analysed by double IF using antibodies to YFP and CCK or GABA in the hypothalamus. Quantification was expressed in percentages (n=3, mean±s.d.). (c) Body weight analysis (male mice). Mutants are significantly heavier than controls starting at 4 M of age (1.5 M,n=12 and 13; 3 M, bothn=12; 4 M,n=9 and 11; 5 M,n=13 and 17; 7.5 M,n=5 and 7; 11 M,n=6 and 8, forTrkbCck-KOand controls, respectively. Values are mean±s.e.m.). (d) Visible size discrepancy betweenTrkbCck-KOand control male mice, including fat pad mass. (e) Body composition determined by NMR at 3 M and 9 M. Old but not youngTrkbCck-KOmice show increased FM but no changes in FFM (9 M, FM,TrkbCck-KO, 12.37±0.96 g (n=5) versus 5.54±0.86 (n=6),P=0.0005, unpaired Student’st-test; FFM,TrkbCck-KO, 31.37±0.87 g (n=5) versus 29.08±1.33 (n=6); 3 M, FM,TrkbCck-KO, 4.16±0.86 g (n=4) versus 2.18±0.19 (n=4),P=0.06, unpaired Student’st-test; FFM,TrkbCck-KO, 24.74±0.96 g (n=4) versus 23.84±0.42 (n=4); mean±s.e.m. (f) Light and dark phases average food intake (2 M,n=4 for all); (8 M,n=6 for all), mean±s.e.m. (g) Similar cumulative food intake observed over 3 weeks for 3 MTrkbCck-KOand controls (n=6 for all; mean±s.e.m.). (h) Average daily food intake over 6 days on SC and HFD (third week is shown) (two-way ANOVA, diet effect: F(1,8)=24.9,P=0.001, Fisher’s PLSDP=0.001; genotype effect, diet*genotype effect were not significant). This experiment was replicated on two independent mouse cohorts. Scale bars, (a) 500 μm; (b) 50 μm. Figure 1: Trkb Cck-KO mice are obese but show no signs of hyperphagia. ( a ) Adult brain section of BAC-Cck-Cre tg/+ ; R26R-EYFP tg/+ stained with G(Y)FP-specific antibodies (Abs). Cre -mediated EYFP expression is detected in the hypothalamus (HY), cortical layers IV and V (CX) and hippocampus (H). ( b ) Cellular specificity of Cre -mediated recombination was analysed by double IF using antibodies to YFP and CCK or GABA in the hypothalamus. Quantification was expressed in percentages ( n =3, mean±s.d.). ( c ) Body weight analysis (male mice). Mutants are significantly heavier than controls starting at 4 M of age (1.5 M, n =12 and 13; 3 M, both n =12; 4 M, n =9 and 11; 5 M, n =13 and 17; 7.5 M, n =5 and 7; 11 M, n =6 and 8, for Trkb Cck-KO and controls, respectively. Values are mean±s.e.m.). ( d ) Visible size discrepancy between Trkb Cck-KO and control male mice, including fat pad mass. ( e ) Body composition determined by NMR at 3 M and 9 M. Old but not young Trkb Cck-KO mice show increased FM but no changes in FFM (9 M, FM, Trkb Cck-KO , 12.37±0.96 g ( n =5) versus 5.54±0.86 ( n =6), P =0.0005, unpaired Student’s t -test; FFM, Trkb Cck-KO , 31.37±0.87 g ( n =5) versus 29.08±1.33 ( n =6); 3 M, FM, Trkb Cck-KO , 4.16±0.86 g ( n =4) versus 2.18±0.19 ( n =4), P =0.06, unpaired Student’s t -test; FFM, Trkb Cck-KO , 24.74±0.96 g ( n =4) versus 23.84±0.42 ( n =4); mean±s.e.m. ( f ) Light and dark phases average food intake (2 M, n =4 for all); (8 M, n =6 for all), mean±s.e.m. ( g ) Similar cumulative food intake observed over 3 weeks for 3 M Trkb Cck-KO and controls ( n =6 for all; mean±s.e.m.). ( h ) Average daily food intake over 6 days on SC and HFD (third week is shown) (two-way ANOVA, diet effect: F(1,8)=24.9, P =0.001, Fisher’s PLSD P =0.001; genotype effect, diet*genotype effect were not significant). This experiment was replicated on two independent mouse cohorts. Scale bars, ( a ) 500 μm; ( b ) 50 μm. Full size image The BAC-Cck-Cre line was then crossed to a Trkb floxed line [29] to specifically delete Trkb from CCK neurons. Deletion of Trkb was verified by western blot (WB) on lysates from cortical and hypothalamic tissues of Trkb Cck-KO mice and controls ( Supplementary Fig. 2a ), and further validated by in situ hybridization combined with immunofluorescence (IF) ( Supplementary Fig. 2b ). These confirmed the specificity and successful inactivation of Trkb in CCK neurons. CCK levels in the brain were not altered by the BAC transgene or the deletion of Trkb ( Supplementary Fig. 2c ). Age-dependent obesity without hyperphagia in Trkb Cck-KO mice Trkb Cck-KO mice develop an age-dependent obesity evident around 4 months (4 M) of age in male ( Fig. 1c,d ), and female mice (5 M Trkb Cck-KO 33.8±1.2 g ( n =17) versus control 26.9±0.8 g ( n =13), P =0.0001, unpaired Student’s t -test, mean±s.e.m.). Analysis of body composition of young (3 M) and old (9 M) male mice by nuclear magnetic resonance (NMR) revealed significant increase in fat mass (FM) but not in fat-free mass (FFM) in 9 M Trkb Cck-KO mutants ( Fig. 1e ). Mouse models carrying a Bdnf or Trkb deficiency exhibit obesity due to hyperphagia [15] , [17] . Trkb hypomorphic mice also have an altered daily pattern of food intake [14] . No changes were detected in the circadian rhythm, or the cumulative amount of food intake in Trkb Cck-KO mutants or controls at either 2 M or 8 M of age ( Fig. 1f,g and Supplementary Fig. 3a ). Despite this, mutants gained significantly more weight ( Supplementary Fig. 3b,c ). Mice subjected to a high fat diet (HFD) decrease their food intake accordingly. Trkb Cck-KO mice on a HFD alter their food intake in a normal manner ( Fig. 1h and Supplementary Fig. 3d,e ). Surprisingly, and in contrast to all published models of Bdnf and/or Trkb deficiency, Trkb Cck-KO mice are not hyperphagic, indicating that their obese phenotype is due to another mechanism. Signs of chronic hypercortisolism in Trkb Cck-KO mice Abdominal obesity has been associated with altered HPA axis activity, elevated glucocorticoid levels and reduced ability of cortisol to suppress its own secretion; all common features of CS [30] . CORT is secreted in hourly pulses with the lowest level at the beginning of the rest period (for rodents in the morning) and the highest level at the beginning of the active period (for rodents in the evening) [31] . Serum ACTH and CORT measurements taken at 08:00 and at 16:00 in 5 M animals showed significantly elevated ACTH in Trkb Cck-KO mice compared with controls at both time points ( Fig. 2a ). In contrast to basal CORT levels, afternoon CORT levels were significantly elevated in 5 M Trkb Cck-KO mice ( Fig. 2b ), demonstrating increased activity of the HPA axis. 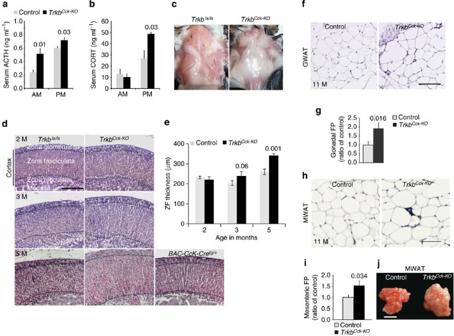Figure 2: HPA axis hyperactivity and signs of chronic hypercortisolism. (a,b) Serum ACTH and CORT levels, morning (AM) and afternoon (PM), were measured by EIA in 5-month-old animals. (a) ACTH AM levels (TrkbCck-KO0.514±0.077 (n=4) versus control 0.240±0.035 ng ml−1(n=5),P=0.01); ACTH PM levels (TrkbCck-KO0.718±0.043 (n=4) versus control 0.601±0.024 ng ml−1(n=5),P=0.03). (b) CORT AM levels (TrkbCck-KO10.3±3.1 (n=4) versus control 13.1±4.2 ng ml−1(n=4),P=0.30); CORT PM levels (TrkbCck-KO48.7±1.8 ng ml−1(n=4) versus control 27.1±6.9 ng ml−1(n=5),P=0.03); values are mean±s.e.m. Hormone measurements were replicated 2–3 times. (c) Increased fat accumulations in the shoulder-neck region ofTrkbCck-KOmice compared with control littermates. (d) Representative haematoxylin/eosin-stained adrenal section images ofTrkbCck-KOfemale mice and littermate controls at 2, 3 and 5 M of age. (e) Average thickness of the ZF in femaleTrkbCck-KOmice compared with controls (2 M,TrkbCck-KO221.1±15.1 versus control 231.7±6.6,n=2/2; 3 M,TrkbCck-KO239.5±20.9 versus control 204.0±11.2,n=3/3,P=0.006; 5 M,TrkbCck-KO341.5±9.3 versus control 260.5±13.7,n=3/3,P=0.001; values are mean±s.d. (f,h) Representative haematoxylin/eosin-stained gonadal and mesenteric white adipose tissue section images (GWAT, MWAT) at 11 M showing enlarged adipocytes inTrkbCck-KOmice. (g,i) GWAT and MWAT weight normalized to body weight as ratio of the control cohort.TrkbCck-KOmice have significantly more adipose tissue (GWAT,TrkbCck-KO, 1.92±0.32 g (n=9) versus control 1.00±0.18 (n=11),P=0.016; MWAT,TrkbCck-KO, 1.53±0.21 g (n=9) versus control 1.00±0.13 (n=11),P=0.034; values are mean±s.e.m.). (j) The increase in adipose tissue inTrkbCck-KOmutants is apparent even in freshly dissected MWAT (whiter) indicating increased incorporation of lipids.Pvalues by unpaired Student’st-test. Scale bars, (d) 200 μm; (f,h) 100 μm; (i) 1 cm. Figure 2: HPA axis hyperactivity and signs of chronic hypercortisolism. ( a , b ) Serum ACTH and CORT levels, morning (AM) and afternoon (PM), were measured by EIA in 5-month-old animals. ( a ) ACTH AM levels ( Trkb Cck-KO 0.514±0.077 ( n =4) versus control 0.240±0.035 ng ml −1 ( n =5), P =0.01); ACTH PM levels ( Trkb Cck-KO 0.718±0.043 ( n =4) versus control 0.601±0.024 ng ml −1 ( n =5), P =0.03). ( b ) CORT AM levels ( Trkb Cck-KO 10.3±3.1 ( n =4) versus control 13.1±4.2 ng ml −1 ( n =4), P =0.30); CORT PM levels ( Trkb Cck-KO 48.7±1.8 ng ml −1 ( n =4) versus control 27.1±6.9 ng ml −1 ( n =5), P =0.03); values are mean±s.e.m. Hormone measurements were replicated 2–3 times. ( c ) Increased fat accumulations in the shoulder-neck region of Trkb Cck-KO mice compared with control littermates. ( d ) Representative haematoxylin/eosin-stained adrenal section images of Trkb Cck-KO female mice and littermate controls at 2, 3 and 5 M of age. ( e ) Average thickness of the ZF in female Trkb Cck-KO mice compared with controls (2 M, Trkb Cck-KO 221.1±15.1 versus control 231.7±6.6, n =2/2; 3 M, Trkb Cck-KO 239.5±20.9 versus control 204.0±11.2, n =3/3, P =0.006; 5 M, Trkb Cck-KO 341.5±9.3 versus control 260.5±13.7, n =3/3, P =0.001; values are mean±s.d. ( f , h ) Representative haematoxylin/eosin-stained gonadal and mesenteric white adipose tissue section images (GWAT, MWAT) at 11 M showing enlarged adipocytes in Trkb Cck-KO mice. ( g , i ) GWAT and MWAT weight normalized to body weight as ratio of the control cohort. Trkb Cck-KO mice have significantly more adipose tissue (GWAT, Trkb Cck-KO , 1.92±0.32 g ( n =9) versus control 1.00±0.18 ( n =11), P =0.016; MWAT, Trkb Cck-KO , 1.53±0.21 g ( n =9) versus control 1.00±0.13 ( n =11), P =0.034; values are mean±s.e.m.). ( j ) The increase in adipose tissue in Trkb Cck-KO mutants is apparent even in freshly dissected MWAT (whiter) indicating increased incorporation of lipids. P values by unpaired Student’s t -test. Scale bars, ( d ) 200 μm; ( f , h ) 100 μm; ( i ) 1 cm. Full size image Diseases of chronic hypercortisolism such as CS are associated with fat accumulation in the shoulder-neck region and with hypertrophy of the CORT-producing cells in the adrenal cortex (zona fasciculata (ZF)) [32] . Analysis of the shoulder/neck region indeed revealed increased fat accumulation in Trkb Cck-KO mice compared with controls ( Fig. 2c ). Examination of the adrenal cortex ZF thickness at 2, 3 and 5 M of age revealed a clear trend of hypertrophy of this region in Trkb Cck-KO mice starting at 3 M, and becoming highly significant by 5 M compared with controls ( Fig. 2d,e ). Therefore, Trkb Cck-KO mice exhibit chronic hypercortisolism caused by hyperactivity of the HPA axis. Chronic high glucocorticoid levels can lead to accumulation of adipose tissue and visceral obesity as seen in Cushing’s patients. To assess whether the observed weight gain in Trkb Cck-KO mice was due to increased adiposity and was depot specific, we first examined two major visceral fat pads: mesenteric and gonadal white adipose tissue (WAT). The mass of each was significantly increased in Trkb Cck-KO male and female mice compared with controls ( Fig. 2f–j ). In contrast, similar amounts of interscapular brown adipose tissue (BAT) deposits were found ( Supplementary Fig. 4a–c ). BAT regulates thermogenesis via the mitochondrial uncoupling protein-1. No significant differences in uncoupling protein-1 expression by immunohistochemistry (IHC) and WB of dissected BAT were observed ( Supplementary Fig. 4d–g ) supporting the lack of involvement of altered thermogenesis in the obesity phenotype. Mice carrying only the Cre transgene did not show significant changes compared with wild-type littermates when tested for signs of hypercortisolism at the critical stages ( Supplementary Fig. 5 , and Supplementary Table 1 ). Together, these results demonstrate that deletion of Trkb from CCK neurons influences HPA axis activity and leads to mild mature-onset obesity with increased WAT accumulation. EE is not impaired in Trkb Cck-KO mice Energy balance is modulated by food intake and energy expenditure (EE). We have shown that Trkb Cck-KO mice show a similar rate of food intake compared with controls and yet develop age-dependent obesity. We next evaluated EE and activity. No differences were observed in oxygen consumption (VO 2 ), carbon dioxide production (VCO 2 ) rates, respiratory exchange ratio (VO 2 : control 3,490.6±70.4 versus mutant 3,397.1±38.0 ml h −1 kg −1 (lean mass), P =0.265; VCO 2 : control 3,274.0±59.1 versus mutant 3,113.5±47.5 ml h −1 kg −1 (lean mass), P =0.06; respiratory exchange ratio: control 0.935±0.005 versus mutant 0.914±0.010 VCO 2 /VO 2 , P =0.9; n =7, for both groups, 8.5 M of age, unpaired Student’s t -test, mean±s.e.m.) or EE between control and obese Trkb Cck-KO mice either in the light or dark phase ( Supplementary Fig. 6a,b ). Home cage activity, instead, revealed a normal circadian rhythm at 2 M of age ( Supplementary Fig. 7a,b ), but a significant increase during the dark phase in 8-month-old obese mutants compared with controls ( Supplementary Fig. 7c,d ). Anxiety-like behaviour, assessed by the open field (OF) and the elevated plus maze, was found to be equivalent in all groups and ages ( Supplementary Fig. 8a–c ). Thus, the increased weight gain and adipose accumulation in Trkb Cck-KO mice is not associated with a decrease in locomotion, or with decreased EE. Chronic hypercortisolism leads to glucose intolerance Leptin and insulin, hormones produced by adipocytes and the pancreas, respectively, have both been implicated in the control of body weight. However, their modes of action are different [33] . Normal levels of serum leptin and insulin were found in 2.5 M Trkb Cck-KO mice fed standard chow (SC) compared with controls ( Fig. 3a,c ). Older obese animals, however, had significant elevated levels of serum leptin and insulin ( Fig. 3b,d ). In addition, the aged Trkb Cck-KO mice had impaired glucose tolerance ( Fig. 3e–f ), and a significant increase in liver mass, and hepatic lipid stores compared with controls ( Fig. 3g–i ). These results suggest that chronic hypercortisolism leads to an age-dependent obesity associated with glucose intolerance and fatty liver, resembling Cushing’s patients. 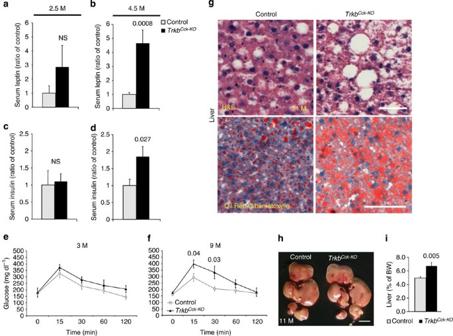Figure 3: Consequences of corticosteroid induced obesity inTrkbCck-KO. (a,b) Serum leptin levels in young-lean (a) and older-obese (b)TrkbCck-KOand controls measured by EIA.TrkbCck-KO(ratio of control, 2.5 M,TrkbCck-KO, 2.85±1.59 (n=3) versus control 1.00±0.85 (n=3); mean±s.d.; 4.5 M,TrkbCck-KO, 4.65±0.95 (n=6) versus control 1.00±0.13 (n=8),P=0.0008, unpaired Student’st-test, mean±s.e.m.). (c,d) Serum insulin levels in young-lean (c) and old-obese (d)TrkbCck-KOand controls measured by EIA.TrkbCck-KO(ratio of control, 2.5 M,TrkbCck-KO, 1.10±0.24 (n=3) versus control 1.00±0.46 (n=3), mean±s.d.); 4.5 M,TrkbCck-KO, 1.87±0.30 (n=4) versus control 1.00±0.19 (n=7),P=0.027, unpaired Student’st-test, mean±s.e.m.). Hormone measurements were replicated 2–3 times. (e,f) Glucose tolerance test in young (e) and old obese (f)TrkbCck-KOand control mice on SC. Glucose (mg dl−1) at 3 M (n=3/4) (0 min,TrkbCck-KOversus controlP=0.9; 15 min,TrkbCck-KOversus controlP=0.4; 30 min,TrkbCck-KOversus controlP=0.2; 60 min,TrkbCck-KOversus controlP=0.4; 120 min,TrkbCck-KOversus controlP=0.1); at 9 M (n=5/6) (0 min,TrkbCck-KOversus controlP=0.3; 15 min,TrkbCck-KOversus controlP=0.04; 30 min,TrkbCck-KOversus controlP=0.03; 60 min,TrkbCck-KOversus controlP=0.1; 120 min,TrkbCck-KOversus controlP=0.8,Pvalues by unpaired Student’st-test. All values are mean±s.e.m.). (g) Liver sections of 11-month-old mice stained with haematoxylin/eosin (upper panels), and Oil-Red-O (lower panels).TrkbCck-KOmice show increased lipid accumulation inTrkbCck-KOmice compared with controls. (h,i) The increase in liver fat content in oldTrkbCck-KOmutants is apparent even in freshly dissected liver (liver weight expressed as % of body weight (BW),TrkbCck-KO, 6.7±0.5% (n=3) versus control 4.9±0.2 (n=3),P=0.005, unpaired Student’st-test, values are mean±s.d.). Livers were analysed in two independent mouse cohorts. Scale bars: (g) upper panel, 50 μm; lower panel, 100 μm; (h) 1 cm. Figure 3: Consequences of corticosteroid induced obesity in Trkb Cck-KO . ( a , b ) Serum leptin levels in young-lean ( a ) and older-obese ( b ) Trkb Cck-KO and controls measured by EIA. Trkb Cck-KO (ratio of control, 2.5 M, Trkb Cck-KO , 2.85±1.59 ( n =3) versus control 1.00±0.85 ( n =3); mean±s.d. ; 4.5 M, Trkb Cck-KO , 4.65±0.95 ( n =6) versus control 1.00±0.13 ( n =8), P =0.0008, unpaired Student’s t -test, mean±s.e.m.). ( c , d ) Serum insulin levels in young-lean ( c ) and old-obese ( d ) Trkb Cck-KO and controls measured by EIA. Trkb Cck-KO (ratio of control, 2.5 M, Trkb Cck-KO , 1.10±0.24 ( n =3) versus control 1.00±0.46 ( n =3), mean±s.d. ); 4.5 M, Trkb Cck-KO , 1.87±0.30 ( n =4) versus control 1.00±0.19 ( n =7), P =0.027, unpaired Student’s t -test, mean±s.e.m.). Hormone measurements were replicated 2–3 times. ( e , f ) Glucose tolerance test in young ( e ) and old obese ( f ) Trkb Cck-KO and control mice on SC. Glucose (mg dl −1 ) at 3 M ( n =3/4) (0 min, Trkb Cck-KO versus control P =0.9; 15 min, Trkb Cck-KO versus control P =0.4; 30 min, Trkb Cck-KO versus control P =0.2; 60 min, Trkb Cck-KO versus control P =0.4; 120 min, Trkb Cck-KO versus control P =0.1); at 9 M ( n =5/6) (0 min, Trkb Cck-KO versus control P =0.3; 15 min, Trkb Cck-KO versus control P =0.04; 30 min, Trkb Cck-KO versus control P =0.03; 60 min, Trkb Cck-KO versus control P =0.1; 120 min, Trkb Cck-KO versus control P =0.8, P values by unpaired Student’s t -test. All values are mean±s.e.m.). ( g ) Liver sections of 11-month-old mice stained with haematoxylin/eosin (upper panels), and Oil-Red-O (lower panels). Trkb Cck-KO mice show increased lipid accumulation in Trkb Cck-KO mice compared with controls. ( h , i ) The increase in liver fat content in old Trkb Cck-KO mutants is apparent even in freshly dissected liver (liver weight expressed as % of body weight (BW), Trkb Cck-KO , 6.7±0.5% ( n =3) versus control 4.9±0.2 ( n =3), P =0.005, unpaired Student’s t -test, values are mean±s.d.). Livers were analysed in two independent mouse cohorts. Scale bars: ( g ) upper panel, 50 μm; lower panel, 100 μm; ( h ) 1 cm. Full size image Impaired inhibition of PVN CRH neurons causes HPA axis hyperactivity We have shown that Trkb deletion in CCK neurons induces hyperactivity of the HPA axis. In order to determine whether TrkB signalling regulates HPA axis activity at the peripheral or central level, we examined Cre -mediated YFP expression in the anterior pituitary and adrenals of BAC-Cck-Cre mice crossed to the R26R-YFP reporter line. Trkb is known to be expressed in the anterior pituitary [34] , but not in the adrenal cortex [35] . We observed only single scattered YFP-positive cells in the anterior pituitary ( Supplementary Fig. 1e ), and in the cortex of the adrenal medulla. This suggests that the HPA axis hyperactivity found in Trkb Cck-KO mice might be due to central changes in PVN neuronal activity. Trkb is expressed in all hypothalamic nuclei [36] , and Cre -mediated YFP expression in the hypothalamus of BAC-Cck-Cre mice is high ( Supplementary Fig. 1b ). We therefore investigated neuronal markers of PVN activity: Crh , Avp and pro-enkephalin ( Penk) ( Fig. 4a–f ). Avp is co-expressed with Crh in parvocellular neurons, co-secreted with CRH upon hypothalamic stimulation and potentiates the effects of CRH [37] . However, the mechanisms regulating their expression are different [38] . Enkephalin is expressed at very low levels in the PVN and in a nucleus located laterally to the PVN [39] . Its expression in the PVN is detectable only under conditions of elevated HPA axis activity [38] , [40] . In situ hybridization revealed significantly increased Crh and Penk expression in the PVN and increased Penk expression also in the adjacent (ventrolateral/lateral) nucleus in Trkb Cck-KO mice compared with controls. In contrast, Avp expression was significantly decreased ( Fig. 4a–f ). We found a similar pattern of expression by quantitative PCR on tissue punches of the PVN ( Fig. 4g ). Therefore, upregulation of Crh and Penk expression concomitant with increased c-Fos expression is a strong indication of increased activity of parvocellular PVN neurons [38] , [40] . 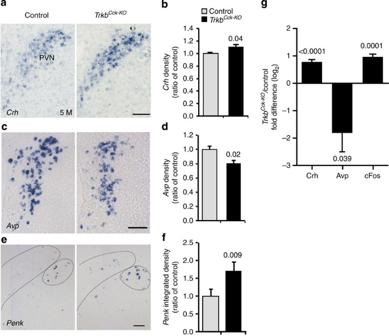Figure 4: Increased HPA axis activity and reduced PVN inhibitory control. (a–e) Images show hypothalamicin situhybridization for several markers of PVN neuronal activity in 5-month-old animals.CrhandAvpexpression highlight the PVN.Penkis expressed at very low levels in the PVN and higher levels in an adjacent nucleus. (a,b) Staining density forCrh(TrkbCck-KO, 1.108±0.043 versus control, 1.00±0.023,P=0.04, unpaired Student’st-test, values are mean±s.e.m.,n=7 per genotype). (c,d)Avp(staining density:TrkbCck-KO, 0.805±0.043 versus control 1.00±0.050,P=0.02, unpaired Student’st-test, values are mean±s.e.m.,n=6 per genotype). (e,f)Penk TrkbCck-KO(integrated density:TrkbCck-KO, 1.717±0.243 versus control 1.000±0.204,P=0.009, unpaired Student’st-test, values are mean±s.d.,n=3 per genotype). (g) Fold difference of gene expression in PVN tissue punches between control andTrkbCck-KOmutants (n=4 per genotype), unpaired Student’st-test, values are mean±s.e.m. Scale bars ina,cande, 100 μm.Avp, arginine vasopressin;Penk, proenkephalin. Figure 4: Increased HPA axis activity and reduced PVN inhibitory control. ( a – e ) Images show hypothalamic in situ hybridization for several markers of PVN neuronal activity in 5-month-old animals. Crh and Avp expression highlight the PVN. Penk is expressed at very low levels in the PVN and higher levels in an adjacent nucleus. ( a , b ) Staining density for Crh ( Trkb Cck-KO , 1.108±0.043 versus control, 1.00±0.023, P =0.04, unpaired Student’s t -test, values are mean±s.e.m., n =7 per genotype). ( c , d ) Avp (staining density: Trkb Cck-KO , 0.805±0.043 versus control 1.00±0.050, P =0.02, unpaired Student’s t -test, values are mean±s.e.m., n =6 per genotype). ( e , f ) Penk Trkb Cck-KO (integrated density: Trkb Cck-KO , 1.717±0.243 versus control 1.000±0.204, P =0.009, unpaired Student’s t -test, values are mean±s.d., n =3 per genotype). ( g ) Fold difference of gene expression in PVN tissue punches between control and Trkb Cck-KO mutants ( n =4 per genotype), unpaired Student’s t -test, values are mean±s.e.m. Scale bars in a , c and e , 100 μm. Avp , arginine vasopressin; Penk , proenkephalin. Full size image Previous reports have demonstrated that an increase in glucocorticoid levels induces activation of GR, and a concurrent increase of the expression/activity of proteins in the MAPK signalling pathway, both in vivo (in the hippocampus) and in vitro (in cell lines) [41] . We had technical difficulties to perform biochemistry using only hypothalamic-targeted CCK neurons, which is a small population, we therefore performed WB analysis of total hypothalamic cell lysates. Considering that this would also include neurons expressing GR and MAPK/PKC in other hypothalamic (non-CCK) cells, it is not surprising that this experiment did not reveal significantly higher activation of ERK and PKC (see ratio of phosphorylated protein/total protein) ( Supplementary Fig. 9a,b , and Supplementary Table 2 ). However, the findings that Crh expression in the PVN is not suppressed, despite elevated glucocorticoid levels, support the hypothesis of impaired central glucocorticoid feedback inhibition in Trkb Cck-KO mice. We next asked how TrkB signalling in GABAergic CCK neurons could influence the activity of PVN-CRH neurons. A ring of inhibitory neurons located around the PVN, residing in the peri-PVN, the medial-dorsal region of the anterior hypothalamic nucleus (AHN) and the dorsomedial nucleus of the hypothalamus (DMH), has been described to integrate glutamatergic and GABAergic input from limbic areas, and to modulate HPA axis activity [8] ( Fig. 5a ). Detailed analysis of the recombination pattern in the BAC-Cck-Cre hypothalamic region revealed that only a few cells in the PVN were YFP-positive, whereas most of the YFP-positive cells clustered in the dorso-medial part of the AHN (peri-PVN), and in the medial preoptic area. In caudal sections, this cluster was found more laterally to the PVN, in particular in the DMH ( Fig. 5b , and Supplementary Fig. 1b ). Therefore, most of the CCK-YFP cells in the hypothalamus of the BAC-Cck-Cre line are part of the ring of inhibitory neurons. CCK-YFP immunoreactivity in these hypothalamic neurons co-localizes with the GR ( Fig. 5c,d ). Approximately 80% of the YFP-positive neurons in the peri-PVN and AHN also co-expressed GR in both Trkb Cck-KO mutants and controls ( Fig. 5e ), suggesting that the absence of TrkB signalling in these neurons does not affect their survival ( Fig. 5d,e ). Analysis of presynaptic GABAergic terminals on CRH-positive PVN neurons by the vesicular GABA transporter (VGAT) immunoreactivity found a non-significant decrease in VGAT+ terminals in Trkb Cck-KO mutants ( Fig. 5f,g ). However, presynaptic GABAergic terminals identified by VGAT immunoreactivity include, but are not exclusive for, CCK+ neurons located around the PVN. Therefore, to specifically analyse hypothalamic CCK fibres projecting to and innervating the PVN-CRH+ neurons, we assessed CCK-YFP terminals to the PVN and found a significantly reduced density of these fibres in Trkb Cck-KO mutants compared with controls ( Fig. 6a,b ). This was accompanied by a significant decrease in MAPKs activation specifically in the PVN ( Fig. 6c,d ). These results suggest reduced inhibitory tone over the PVN CRH neurons by the local CCK neurons lacking TrkB signalling. 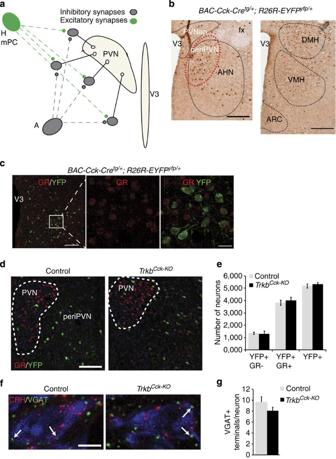Figure 5: Hypothalamic CCK-YFP+ cells and the inhibitory neurons ring. (a) Schematic representation showing that afferent limbic projections, for example, from the hippocampus (H), the medial prefrontal cortex (mPC) and the amygdala (A), do not contact the medial parvocellular neurons (PVN) directly; they contact local GABAergic interneurons that in turn innervate the PVN (adapted from Hermanet al.8). (b) Coronal sections through the hypothalamus of an adultBAC-Cck-Cretg/+;R26R-EYFPyfp/+mouse brain stained with anti-G(Y)FP, showing EYFP expressing cells in the hypothalamic nuclei. (c) AdultBAC-Cck-Cretg/+;R26R-EYFyfp/+mouse hypothalamic section containing the AHN, and stained by double IF with antibodies to the GR and EYFP. Most of the EYFP-expressing neurons also express GR. (d) Representative images of hypothalamic sections stained with anti-(Y)GFP (green), anti-GR (red) and DAPI (blue) from controls (BAC-Cck-Cretg/+;Trkb+/+;R26R-EYFPyfp/+) and mutants (TrkbCck-KO;R26R-EYFyfp/+). (e) Number of YFP-positive neurons in the peri-PVN and AHN and co-expression of GR. YFP+(TrkbCck-KO, 5311.5±171.7 versus control 5196.7±164.9,P=0.6). YFP+GR+(TrkbCck-KO, 4016.7±260 versus control 3838.7±211.5,P=0.6). YFP+GR−(TrkbCck-KO, 1294.9±252 versus control 1,358±86,P=0.8); unpaired Student’st-test, values are mean±s.e.m;n=4 per genotype. (f) Representative images of PVN sections stained with VGAT (green), CRH (red) and Neurotrace fluorescent Nissl (blue), arrows indicate typical VGAT terminals. (g) Quantification of VGAT-positive terminals on CRH-positive neurons in the PVN (TrkbCck-KO, 8.0±0.7 versus control 9.6±1.1,P=0.26; unpaired Student’st-test, values are mean±s.e.m.,n=4 per genotype). PVNap, anterior parvocellular part of the hypothalamic PVN; DMH, dorsomedial nucleus; VMH, ventromedial nucleus; ARC, arcuate nucleus; fx, fornix; V3, third ventricle. Scale bars: (b) 200 μm; (c) 100 μm; (left panel), 20 μm (right panel); (d) 100 μm; (f) 5 μm. Figure 5: Hypothalamic CCK-YFP+ cells and the inhibitory neurons ring. ( a ) Schematic representation showing that afferent limbic projections, for example, from the hippocampus (H), the medial prefrontal cortex (mPC) and the amygdala (A), do not contact the medial parvocellular neurons (PVN) directly; they contact local GABAergic interneurons that in turn innervate the PVN (adapted from Herman et al. [8] ). ( b ) Coronal sections through the hypothalamus of an adult BAC-Cck-Cre tg/+ ;R26R-EYFP yfp/+ mouse brain stained with anti-G(Y)FP, showing EYFP expressing cells in the hypothalamic nuclei. ( c ) Adult BAC-Cck-Cre tg/+ ;R26R-EYF yfp/+ mouse hypothalamic section containing the AHN, and stained by double IF with antibodies to the GR and EYFP. Most of the EYFP-expressing neurons also express GR. ( d ) Representative images of hypothalamic sections stained with anti-(Y)GFP (green), anti-GR (red) and DAPI (blue) from controls ( BAC-Cck-Cre tg/+ ;Trkb +/+ ;R26R-EYFP yfp/+ ) and mutants ( Trkb Cck-KO ;R26R-EYF yfp/+ ). ( e ) Number of YFP-positive neurons in the peri-PVN and AHN and co-expression of GR. YFP + ( Trkb Cck-KO , 5311.5±171.7 versus control 5196.7±164.9, P =0.6). YFP + GR + ( Trkb Cck-KO , 4016.7±260 versus control 3838.7±211.5, P =0.6). YFP + GR − ( Trkb Cck-KO , 1294.9±252 versus control 1,358±86, P =0.8); unpaired Student’s t -test, values are mean±s.e.m; n =4 per genotype. ( f ) Representative images of PVN sections stained with VGAT (green), CRH (red) and Neurotrace fluorescent Nissl (blue), arrows indicate typical VGAT terminals. ( g ) Quantification of VGAT-positive terminals on CRH-positive neurons in the PVN ( Trkb Cck-KO , 8.0±0.7 versus control 9.6±1.1, P =0.26; unpaired Student’s t -test, values are mean±s.e.m., n =4 per genotype). PVNap, anterior parvocellular part of the hypothalamic PVN; DMH, dorsomedial nucleus; VMH, ventromedial nucleus; ARC, arcuate nucleus; fx, fornix; V3, third ventricle. Scale bars: ( b ) 200 μm; ( c ) 100 μm; (left panel), 20 μm (right panel); ( d ) 100 μm; ( f ) 5 μm. 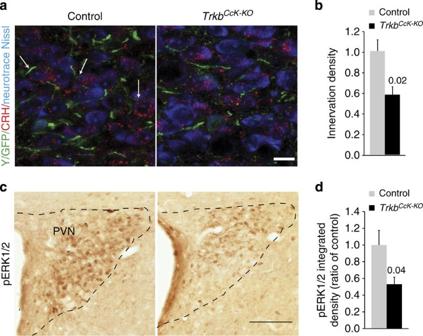Figure 6: Reduced CCK-YFP+ fibres targeting CRH-PVN neurons. (a,b) PVN from controls (BAC-Cck-Cretg/+; Trkb+/+; R26R-EYFPyfp/+) and mutant (TrkbCck-KO; R26R-EYFyfp/+) mice stained for YFP (green), CRH (red) and Neurotrace Nissl (blue). YFP+ processes can be found in the vicinity of CRH+ neurons (white arrows). Mutants show decreased YFP+ fibres (innervation density, ratio: control 1.000±0.114 (n=4); mutant 0.577±0.082 (n=4);P=0.02, unpaired Student’st-test, values are mean±s.e.m.). Scale bar, 10 μm. (c,d) Reduced MAPK signalling in the PVN ofTrkbCck-KOmice. PVN sections from controls andTrkbCck-KOmutants were immunostained with pERK1/2 antibodies and integrated staining density was quantified. Mutants showed decreased integrated staining density in the PVN compared with controls (ratio, mutants 0.531±0.083 versus 1.000±0.174,n=5,P=0.04, unpaired Student’st-test, values are mean±s.e.m.). Scale bar, 100 μm. Full size image Figure 6: Reduced CCK-YFP+ fibres targeting CRH-PVN neurons. ( a , b ) PVN from controls ( BAC-Cck-Cre tg/+ ; Trkb +/+ ; R26R-EYFP yfp/+ ) and mutant ( Trkb Cck-KO ; R26R-EYF yfp/+ ) mice stained for YFP (green), CRH (red) and Neurotrace Nissl (blue). YFP+ processes can be found in the vicinity of CRH+ neurons (white arrows). Mutants show decreased YFP+ fibres (innervation density, ratio: control 1.000±0.114 ( n =4); mutant 0.577±0.082 ( n =4); P =0.02, unpaired Student’s t -test, values are mean±s.e.m.). Scale bar, 10 μm. ( c , d ) Reduced MAPK signalling in the PVN of Trkb Cck-KO mice. PVN sections from controls and Trkb Cck-KO mutants were immunostained with pERK1/2 antibodies and integrated staining density was quantified. Mutants showed decreased integrated staining density in the PVN compared with controls (ratio, mutants 0.531±0.083 versus 1.000±0.174, n =5, P =0.04, unpaired Student’s t -test, values are mean±s.e.m.). Scale bar, 100 μm. Full size image CCK neurons are also present in various other brain regions such as limbic areas, which also play a crucial role in the regulation of HPA axis activity through a multisynaptic process integrated in the hypothalamus by local circuit neurons [8] ( Fig. 5a ). To determine whether ablation of TrkB signalling in CCK neurons in limbic regions would contribute to the observed HPA axis dysfunction in the Trkb Cck-KO mice, we assessed the response of CRH neurons to a psychogenic stressor (restraint stress). The limbic system is well known to regulate the HPA function through this type of stress [5] . Mutant mice subjected to acute restraint stress showed similar levels of serum ACTH and CORT compared with control mice ( Supplementary Fig. 10a,b ), suggesting a normal stress response of the HPA axis in mutants. In summary, deletion of Trkb from CCK local inhibitory neurons impairs inhibitory control over the PVN by reducing GABAergic output of CCK interneurons onto CRH neurons, and causes increased activity of these neurons. Moreover, co-expression of GR in CCK neurons supports a potential role for TrkB signalling in the modulation of central glucocorticoid/GR feedback inhibition. Increased de novo lipogenesis in Trkb Cck-KO mice We then asked whether the hypercortisolism associated with insulin resistance in Trkb Cck-KO mice could affect lipid homeostasis and so fat accumulation. In mammals, the liver is a major site of de novo lipogenesis. Glucocorticoids exert potent actions on lipid homeostasis in human adipose tissue; these effects are dependent upon interactions with insulin, a major regulator of hepatic lipogenesis [42] , [43] . Acetyl-coenzyme-A carboxylase (ACC1) controls fatty acid biosynthesis, and it is expressed mainly in lipogenic tissues such as liver and adipose [44] . ACC1 activity is highly regulated at the expression level and is negatively regulated by phosphorylation at Ser-79 (ref. 45) [45] . We found significantly increased ACC1 protein levels and decreased Ser-79 phosphorylation in livers of Trkb Cck-KO compared with controls ( Fig. 7a,c,d ), indicating increased de novo lipogenesis. GRs are considered to be inactive when dephosphorylated [46] . Liver GR protein levels were reduced in mutants compared with controls, but GR phosphorylation was unaffected relative to its abundance ( Fig. 7b,e–g ) denoting its activity. Interestingly, at 3 M, before obesity was evident, there was already a significant increase of ACC1 levels and GR phosphorylation in liver tissue, but not in WAT, of mutants compared with controls ( Fig. 7h,j,k and Fig. 7i,l–n , and Supplementary Fig. 11b,c ). To test if the increased lipogenesis observed in Trkb Cck-KO mutants was glucocorticoid-dependent we treated old obese (9 M) mutants with a GR antagonist, mifepristone (RU-486). This has been shown to produce clinical and metabolic benefits in Cushing’s patients [47] . After 2 months of treatment, liver GR protein levels and phosphorylation, as well as ACC1 levels, were both significantly reduced in the drug-treated Trkb Cck-KO mutants compared with those vehicle-treated mutants ( Fig. 7a–g ). Analysis of WAT showed a similar downregulation of GR in these groups ( Supplementary Fig. 11a ). Liver fat accumulation was significantly diminished in mifepristone-treated mutants as determined by Oil Red O staining ( Fig. 7o–r ). The effect on WAT accumulation was less evident as the total body weight of mutants did not decrease significantly over the 2-months treatment, but rather their weight stabilized ( Fig. 7u ). These data show that increased de novo lipogenesis in Trkb Cck-KO mutants is likely to account for the fat accumulation observed in these animals, and that the effects are glucocorticoid-dependent. 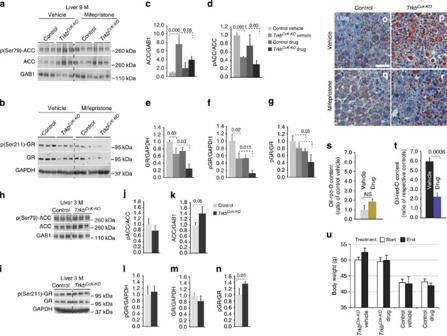Figure 7: Increased lipogenesis inTrkbCck-KOis glucocorticoid-dependent. (a,b) Representative immunoblots of liver lysates from vehicle- and mifepristone-treated animals (9 M,n=3 for mutants and controls of all treatments). (a) WB of ACC and pACC. Loading control, GAB1. (b) WB of GR and pGR. Loading control, GAPDH. (c,d) and (e–g) Quantification of immunoreactivity from WB inaandb, respectively. (c) ACC/GAB1 (ANOVA, genotype: F(1,8)=0.99,P=0.0006; genotype-treatment interaction: F(1,8)=0.79,P=0.016; mutant vehicle versus control vehicle,P=0.006; mutant vehicle versus mutant drug,P=0.05); (d) pACC/ACC (ANOVA, genotype: F(1,8)=0.99,P=0.0005; treatment: F(1,8)=0.58),P=0.038; control vehicle versus mutant vehicle,P=0.0001; mutant vehicle versus mutant drug,P=0.034). (e) GR/GAPDH (ANOVA, genotype: F(1,8)=0.99,P=0.001; treatment: F(1,8)=1.0,P<0.001; control vehicle versus mutant vehicle,P=0.03; mutant vehicle versus mutant drug,P=0.03; (f) pGR/GAPDH (ANOVA, control vehicle versus mutant vehicle,P=0.02; mutant vehicle versus mutant drug,P=0.015; (g) pGR/GR (ANOVA, genotype: F(1,8)=0.92,P=0.005; treatment: F(1,8)=0.68),P=0.02; control vehicle versus mutant vehicle,P=0.2; mutant vehicle versus mutant drug, or control vehicle versus control drug,P=0.05). For all groupsn=3, unpaired Student’st-test. mean±s.d. (h,i) Representative immunoblots of liver lysates from 3-month-old mutants and controls (n=3 for both genotypes). (h) WB of ACC and pACC. Loading control, GAB1. (i) WB for GR and pGR. Loading control, GAPDH. (j,k) and (l–n) Quantification of immunoreactivity from WB inhandi, respectively. (j) pACC/ACC, not significantly different. (k) ACC/GAB1 (mutant vehicle versus control vehicle,P=0.05). (l) pGR/GAPDH and (m) GR/GAPDH, not significantly different. (n) pGR/GR (mutant vehicle versus control vehicle,P=0.05). Unpaired Student’st-test, mean±s.d. WBs were replicated 2–3 times. (Full-length immunoblot images are shown inSupplementary Fig. 13). (o–r) Representative images of liver sections stained with haematoxylin and Oil-Red-O. (s,t) Quantification of Oil-Red-O in livers of vehicle and mifepristone treated control and mutant mice. (s) Control vehicle 1.000±0.435 (n=3) versus control drug 1.834±0.312 (n=5), values were normalized to the mean of the control vehicle group;P=0.163, unpaired Student’s t-test. (t) Mutant groups were normalized to the mean of the respective control group; mutant vehicle 5.936±0.363 (n=3) versus mutant drug 2.221±0.394 (n=6),P=0.0006. Unpaired Student’st-test, mean±s.e.m. (u) Body weight at the beginning of treatment (Start) and in the last week of 8 weeks of mifepristone treatment (End) (control vehiclen=6, control drugn=5, mutant vehiclen=3, mutant drugn=6, mean±s.e.m). Scale bar ino, 50 μm. Figure 7: Increased lipogenesis in Trkb Cck-KO is glucocorticoid-dependent. ( a , b ) Representative immunoblots of liver lysates from vehicle- and mifepristone-treated animals (9 M, n =3 for mutants and controls of all treatments). ( a ) WB of ACC and pACC. Loading control, GAB1. ( b ) WB of GR and pGR. Loading control, GAPDH. ( c , d ) and ( e – g ) Quantification of immunoreactivity from WB in a and b , respectively. ( c ) ACC/GAB1 (ANOVA, genotype: F(1,8)=0.99, P =0.0006; genotype-treatment interaction: F(1,8)=0.79, P =0.016; mutant vehicle versus control vehicle, P =0.006; mutant vehicle versus mutant drug, P =0.05); ( d ) pACC/ACC (ANOVA, genotype: F(1,8)=0.99, P =0.0005; treatment: F(1,8)=0.58), P =0.038; control vehicle versus mutant vehicle, P =0.0001; mutant vehicle versus mutant drug, P =0.034). ( e ) GR/GAPDH (ANOVA, genotype: F(1,8)=0.99, P =0.001; treatment: F(1,8)=1.0, P <0.001; control vehicle versus mutant vehicle, P =0.03; mutant vehicle versus mutant drug, P =0.03; ( f ) pGR/GAPDH (ANOVA, control vehicle versus mutant vehicle, P =0.02; mutant vehicle versus mutant drug, P =0.015; ( g ) pGR/GR (ANOVA, genotype: F(1,8)=0.92, P =0.005; treatment: F(1,8)=0.68), P =0.02; control vehicle versus mutant vehicle, P =0.2; mutant vehicle versus mutant drug, or control vehicle versus control drug, P =0.05). For all groups n =3, unpaired Student’s t -test. mean±s.d. ( h , i ) Representative immunoblots of liver lysates from 3-month-old mutants and controls ( n =3 for both genotypes). ( h ) WB of ACC and pACC. Loading control, GAB1. ( i ) WB for GR and pGR. Loading control, GAPDH. ( j , k ) and ( l – n ) Quantification of immunoreactivity from WB in h and i , respectively. ( j ) pACC/ACC, not significantly different. ( k ) ACC/GAB1 (mutant vehicle versus control vehicle, P =0.05). ( l ) pGR/GAPDH and ( m ) GR/GAPDH, not significantly different. ( n ) pGR/GR (mutant vehicle versus control vehicle, P =0.05). Unpaired Student’s t -test, mean±s.d. WBs were replicated 2–3 times. (Full-length immunoblot images are shown in Supplementary Fig. 13 ). ( o – r ) Representative images of liver sections stained with haematoxylin and Oil-Red-O. ( s , t ) Quantification of Oil-Red-O in livers of vehicle and mifepristone treated control and mutant mice. ( s ) Control vehicle 1.000±0.435 ( n =3) versus control drug 1.834±0.312 ( n =5), values were normalized to the mean of the control vehicle group; P =0.163, unpaired Student’s t- t est. ( t ) Mutant groups were normalized to the mean of the respective control group; mutant vehicle 5.936±0.363 ( n =3) versus mutant drug 2.221±0.394 ( n =6), P =0.0006. Unpaired Student’s t -test, mean±s.e.m. ( u ) Body weight at the beginning of treatment (Start) and in the last week of 8 weeks of mifepristone treatment (End) (control vehicle n =6, control drug n =5, mutant vehicle n =3, mutant drug n =6, mean±s.e.m). Scale bar in o , 50 μm. Full size image The PLCγ-site of TrkB modulates HPA axis activity regulation The TrkB receptor activates different signalling cascades [12] . To assess whether a particular cascade was involved in the regulation of the HPA axis activity, we examined mice carrying a constitutive point mutation at different adaptor sites ( Trkb SHC or Trkb PLC ) [48] . Only heterozygous mutants for each line were analysed as they lack significant peripheral abnormalities and so allow the analysis of phenotypes in the CNS [12] . Although this does not solve the fact that the point mutation will be also in other neurons other than the CCK-positive ones, it is interesting to note that heterozygous Trkb PLC male and female mice showed a mature obesity phenotype similar to that in Trkb Cck-KO mice ( Fig. 8a , shows the data for female mice) (male mice, body weight: 4 M, Trkb PLC/+ 42.81±1.33 g versus Trkb W/+ 33.22±0.869, P <0.0001; 6–7 M, Trkb PLC/+ 51.37±0.946 g versus Trkb W/+ 37.59±0.125, P <0.0001; unpaired Student’s t -test, values are mean±s.e.m., n =4–5 per group analysed). The Trkb SHC heterozygous mutants showed no significant difference in weight compared with control littermates (5–6 M, male mice: Trkb SHC/+ versus Trkb +/+ , P =0.11; female mice: Trkb SHC/+ versus Trkb +/+ , P =0.91; n =4 per group analysed, unpaired Student’s t -test). Morphological analysis of the adrenal cortex exhibited clear hypertrophy and significantly increased thickness of the ZF in Trkb PLC/+ mice ( Fig. 8b,c ). No such hypertrophy was observed in Trkb SHC/+ mice at similar age. Trkb PLC/+ animals (5 M) exhibited also other phenotypes seen in the Trkb Cck-KO mutant mice: increased afternoon ACTH serum levels ( Fig. 8d ), significantly enlarged abdominal fat pad masses ( Fig. 8e ), elevated levels of leptin and insulin ( Fig. 8f ) and increased lipid accumulation in the liver ( Fig. 8g ). No difference was found in the cumulative food intake measured over 3 weeks in 7-month-old Trkb PLC/+ compared with TrkbW /+ controls ( Supplementary Fig. 12a,b ). In conclusion, signalling through the PLCγ-adaptor site of TrkB is capable of regulating HPA axis activity. 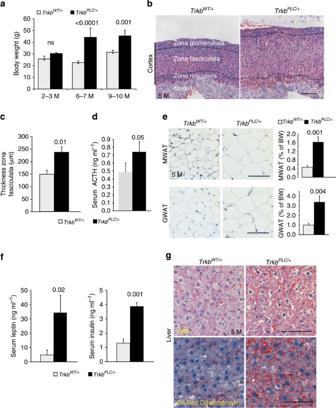Figure 8: The PLCγ-site of TrkB plays a role in HPA axis activity. (a) Body weight of femaleTrkbPLC/+and control (TrkbWT/+) mice (2–3 M,TrkbPLC/+30.25±0.375 versus control 25.54±0.797 g,P=0.17; 6–7 M,TrkbPLC/+44.00±3.9 versus control 22.44±1.0 g,P<0.0001; 9–10 M,TrkbPLC/+45.21±2.3 versus control 31.25±1.2 g,P=0.001; values are mean±s.e.m.,n=4 to 9 per group analysed). (b) Haematoxylin/eosin-stained adrenals of 5-month-oldTrkbPLC/+mice and respective controls (n=3). (c) Average thickness of the ZF inTrkbPLC/+mice compared with controls (female miceTrkbPLC/+238.2±20.0 versus control 148.1±15.8 μm,P=0.01;n=3, values are mean±s.d.). (d) ACTH PM levels (5 M,TrkbPLC/+0.743±0.102 versus control 0.487±0.0477, ng ml−1,P=0.05;n=2/3, values are mean±s.d.). (e) Representative images of haematoxylin/eosin-stained MWAT and GWAT sections and fat pad weight in 5-month-old male mice (MWAT in % of BW,TrkbPLC/+1.63±0.25 versus control 0.46±0.08,P=0.001; GWAT in % of BW,TrkbPLC/+3.40±0.63 versus control 1.00±0.18,P=0.004;n=6, values are mean±s.e.m.). (f) Serum measurements of leptin and insulin (5 M,TrkbPLC/+, leptin 34.4±12.5 versus control 4.8±3.3 ng ml−1,P=0.02; insulin, 3.9±0.4 versus control 1.3±0.3 ng ml−1,P=0.001);n=3, values are mean±s.d. AllPvalues are unpaired Student’st-test. (g) Liver images of 5-month-oldTrkbPLC/+mutants show increased lipid accumulation compared with controls as seen by Oil-Red-O staining. Liver sections stained with haematoxylin/eosin (upper panels), and Oil Red O/haematoxylin (lower panels). All scale bars are 100 μm. Figure 8: The PLCγ-site of TrkB plays a role in HPA axis activity. ( a ) Body weight of female Trkb PLC/+ and control ( Trkb WT/+ ) mice (2–3 M, Trkb PLC/+ 30.25±0.375 versus control 25.54±0.797 g, P =0.17; 6–7 M, Trkb PLC/+ 44.00±3.9 versus control 22.44±1.0 g, P <0.0001; 9–10 M, Trkb PLC/+ 45.21±2.3 versus control 31.25±1.2 g, P =0.001; values are mean±s.e.m., n =4 to 9 per group analysed). ( b ) Haematoxylin/eosin-stained adrenals of 5-month-old Trkb PLC/+ mice and respective controls ( n =3). ( c ) Average thickness of the ZF in Trkb PLC/+ mice compared with controls (female mice Trkb PLC/+ 238.2±20.0 versus control 148.1±15.8 μm, P =0.01; n =3, values are mean±s.d.). ( d ) ACTH PM levels (5 M, Trkb PLC/+ 0.743±0.102 versus control 0.487±0.0477, ng ml −1 , P =0.05; n =2/3, values are mean±s.d.). ( e ) Representative images of haematoxylin/eosin-stained MWAT and GWAT sections and fat pad weight in 5-month-old male mice (MWAT in % of BW, Trkb PLC/+ 1.63±0.25 versus control 0.46±0.08, P =0.001; GWAT in % of BW, Trkb PLC/+ 3.40±0.63 versus control 1.00±0.18, P =0.004; n =6, values are mean±s.e.m.). ( f ) Serum measurements of leptin and insulin (5 M, Trkb PLC/+ , leptin 34.4±12.5 versus control 4.8±3.3 ng ml −1 , P =0.02; insulin, 3.9±0.4 versus control 1.3±0.3 ng ml −1 , P =0.001); n =3, values are mean±s.d. All P values are unpaired Student’s t -test. ( g ) Liver images of 5-month-old Trkb PLC/+ mutants show increased lipid accumulation compared with controls as seen by Oil-Red-O staining. Liver sections stained with haematoxylin/eosin (upper panels), and Oil Red O/haematoxylin (lower panels). All scale bars are 100 μm. Full size image Regulation of the HPA axis activity at the central level is poorly understood, as is a critical neuronal cell-type exerting tonic inhibition over the PVN. We now report that specific deletion of Trkb from CCK neurons disrupts central glucocorticoid negative feedback leading to overt signs of human CS such as hypercortisolism, glucose intolerance and increased lipogenesis associated with an age-dependent obesity. These data therefore provide a critical cell type and a novel mechanism to control HPA axis activity and balance physiological stress responses. It is well established that BDNF-TrkB signalling is required for normal feeding behaviour and control of body weight. Studies involving genetic manipulation of BDNF/TrkB signalling inducing hyperphagia and obesity [13] , [14] , [16] , [17] , and BDNF administration in rodents that reduces food intake [49] , [50] , largely support this view. In contrast, the present genetic manipulation of Trkb uncovers CCK neurons as a critical cellular component of the HPA axis at the central level. Previous reports based on humans and describing a point mutation in the Bdnf locus associated with HPA axis reactivity also support our findings [19] , [20] . HPA axis activity is tightly regulated at the central level; CRH secretion from PVN-parvocellular neurons is strictly controlled by local inhibitory neurons [8] , [9] . The Cre-line used in this study shows recombination in the majority of CCK-GABAergic hypothalamic neurons surrounding the PVN. Deletion of Trkb from these interneurons may therefore impair inhibitory control over PVN-parvocellular neurons by interfering with the integration of the synaptic input from the limbic system. A similar process has been described for the hippocampus [11] . Indeed, increased levels of CORT resulted in Trkb Cck-KO mice being unable to initiate feedback inhibition of Crh expression, supporting an impaired glucocorticoid negative feedback at the central level. This impairment is specific for Crh in the PVN, but not for Avp , whose expression is suppressed in Trkb Cck-KO mice. This is consistent with the theory that Avp and Crh expression are regulated by different mechanisms [38] . The observation of elevated Penk and c-Fos expression, both detectable only under conditions of heightened HPA axis activity, as well as elevated Crh expression, confirms hyperactivity of the PVN [38] , [40] . Chronic hypercortisolism, as seen in CS, leads to increased abdominal adiposity [30] . Our model confirms that chronic exposure to increased glucocorticoid levels is sufficient to induce obesity. Indeed, HPA axis hyperactivity did not affect energy balance through increasing food consumption or EE. However, we did find increased liver de novo lipogenesis, which would account for the accumulation of fat. Glucocorticoids have been shown to exert potent effects on lipid homeostasis in human adipose tissue via interactions with insulin, a major regulator of hepatic lipogenesis [42] , [43] . Blocking GR activity with an antagonist in obese Trkb Cck-KO mice reduced the activity of acetyl-coenzyme-A carboxylase and significantly improved liver fat accumulation. The reduced lipogenesis confirms that obesity in these mice is due to hyperactivity of the HPA axis. Particularly interesting, however, is that manipulation of BDNF/TrkB signalling in CCK interneurons recapitulates primary features of CS. Previous attempts to recapitulate critical features of human CS have met with very little success [51] , [52] , [53] , [54] . The most apparent discrepancy between known forms of human CS, models of chronic hypercortisolism generated previously in rodents and our new model is that hypercortisolism can lead to hyperphagia [55] , and the Trkb Cck-KO mice lack hyperphagia. Exogenous administration of glucocorticoid both in rodents and in humans leads to decreased Crh expression via negative feedback inhibition and therefore the anorexigenic effect of Crh is suppressed [30] resulting in hyperphagia. In our model, instead, hypercortisolism is caused by central dysregulation and impaired glucocorticoid negative feedback inhibition, resulting in increased Crh expression and leaving its anorexigenic effect and food intake regulation intact. Moreover, it has also been shown that chronic exposure to BDNF reduces food intake via the CRH pathway in the PVN [50] . In our model, there is minimal recombination of Trkb in the PVN indicating that BDNF-TrkB signalling regulation of feeding behaviour in the mutants is intact. How does BDNF/TrkB signalling interfere with the glucocorticoid negative feedback in CCK neurons? Genetic dissection of murine GR function has revealed that negative feedback control of the HPA axis, such as repression of Crh synthesis, does not require GR DNA-binding, suggesting a mechanism of repression based on protein–protein interactions, or by cytoplasmic interaction with other proteins [56] . TrkB and GR have been identified in a protein complex in cortical neurons suggesting a possible interaction. This interaction has been shown to enhance BDNF-TrkB signalling through the PLCγ adaptor site [57] . Signalling via TrkB is known to occur predominantly through two adaptor sites, the SHC docking site and the PLCγ docking site [12] . Here we have shown that in vivo a point mutation at the PLCγ docking site ( Trkb PLC ) leads to phenotypes seen in Trkb Cck-KO mice that were not observed in mice carrying a point mutation at the SHC site ( Trkb SHC ). However, we were unable to show an interaction between GR and TrkB by immunoprecipitation of GR, TrkB or PLCγ from naïve or CORT-treated hypothalamic or hippocampal total cell lysates. This may reflect an actual difference between cultures and in vivo systems, or simply that more sensitive techniques would be needed to address this specific question in vivo . This theory, however, is supported by recent work [58] describing crosstalk between GR and TrkB signalling activated-pathways, including activation of PLCγ during aversive memory formation in the rat. The authors were also unable to demonstrate any direct interaction between the two receptors in vivo [58] . In addition, we have also found a significant decrease of projecting CCK-YFP+ fibres associated with CRH neurons in the PVN of mutant mice. This suggests decreased CCK neuronal output onto CRH parvocellular neurons in the mutants, hence reduced inhibitory control over CRH neurons and increased HPA axis activity. We would therefore hypothesize that Trkb deletion in CCK neurons disrupts the communication between TrkB and GR, but also affects CCK projections to the PVN. Consequently, these impair glucocorticoid feedback inhibition, and cause increased responsiveness and hyperactivity of parvocellular PVN neurons. However, a combination of more sophisticated techniques would be required to achieve the spatial resolution that allows to conclude that only the hypothalamic CCK neurons, in the absence of TrkB signalling, are sufficient to disrupt glucocorticoid feedback inhibition at the central level. Nonetheless, this is the first in vivo demonstration, to our knowledge, of a neuronal cell type being pivotal in CNS regulation of HPA axis activity. The identification of signalling via the TrkB PLCγ site gives us an insight into a fundamental pathway involved in glucocorticoid feedback inhibition. Ethics statement All animal procedures at the European Molecular Biology Laboratory (Mouse Biology Unit) conformed to National and International laws and policies (EEC Council Directive 86/609, OJ L 358, 1, 12 December 1987; NIH Guide for the Care and Use of Laboratory Animals, NIH Publication No. 85-23, 1985 revised in 1995); at the University of Edinburgh and the University of Oxford conformed to UK legislation Animals (Scientific procedures) Act 1986. Mouse strains BAC-Cck-Cre strain. A BAC (Clone-ID: RP23-26B6, NCBI Clone Registry) containing the Cck gene was targeted via ET (RecE-RecT)-recombination to insert a Cre-recombinase cassette into the first ATG of the first coding exon (exon 2). The cassette inserted comprised a hybrid intron preceding the Cre- recombinase gene, an internal ribosomal entry site upstream of the beta-galactosidase gene ( LacZ ); the inclusion of LacZ should allow faster identification of transgene expression by X-gal staining; and a neomycin/kanamycin drug-resistance cassette (neo). After successful insertion of the Cre-cassette into the BAC the FRT-flanked neomycin/kanamycin cassette was removed using Flp-recombinase. Circular BAC DNA was injected at 1–2 ng μl −1 into pronuclei of oocytes (CBA/C57 hybrid). TrkB point signalling mutant lines ( Trkb SHC or Trkb PLC and relative control line, Trkb WT ) have been previously described [48] . Trkb Cck-KO mice. The Trkb -floxed ( Trkb lx ) line has been described previously [29] and has been crossed to the BAC-Cck-Cre line to generate the ‘ Trkb Cck-KO ’ ( Trkb lx/lx;Cck-Cretg/+ ) mice. Floxed littermates ( Trkb lx/lx ) without the Cre transgene were used as controls, unless specified. Male and female mice were analysed separately and only combined if comparable. However, to ensure that the transgene did not carry any phenotype, mice carrying only the transgene ( BAC-Cck-Cre tg/+ ) and wild-type control littermates underwent similar analyses ( Supplementary Fig. 5 ). Moreover, no differences were found between wild-type and TrkB floxed animals. Immunoblotting For brain tissues, 3–4-month-old male and female mice were anesthetized with avertin (500 mg kg −1 i.p., Sigma-Aldrich) or sodium pentobarbital (400 mg kg −1 i.p.) and perfused with 1 × PBS. For liver and adipose tissues, mice were culled by cervical dislocation, and tissues snap frozen immediately on dry ice. Tissues were homogenized in 10 volumes (vol/wt) lysis buffer (150 mM NaCl, 50 mM Tris pH 8.0, 1% (vol/vol) NP-40, 0.1% (wt/vol) SDS plus a cocktail of protease and phosphatase inhibitors (Pierce/Thermo Scientific, #88661 and #88667)) with a glass dounce tissue grinder (VWR), followed by mild sonication and centrifugation for 1 h at 20,000 r.p.m. For ACC detection, SDS was increased to 1% (wt/vol) and 4 M Urea was added. Supernatants were subjected to SDS–PAGE and gels blotted onto nitrocellulose membranes (GE healthcare) using a Mini Trans-Blot Cell (Biorad). Membranes were blocked with TBST containing 5% (wt/vol) skimmed milk (Fluka), and probed with specific antibodies ( Supplementary Table 3 ), followed by incubation with HRP-conjugated secondary antibody (1:10,000, Jackson Lab). Bands were visualized by using the SuperSignal West Pico Chemiluminescent Substrate System (Pierce) and BioMax Light Films (Kodak). Histology and IHC Mice (3–4-month-old male and female mice) were perfused with 0.1 M phosphate buffer, pH 7.4, followed by 4% PFA in phosphate buffer. Tissues were dissected, post-fixed overnight in 4% PFA at 4 °C, cryoprotected in 30% (wt/vol) sucrose in Tris-Azide buffer (40 mM Tris, 10 mM phosphate, 0.7% (w/vol) NaCl, 0.05% (w/vol) NaN 3 ) at 4 °C, and frozen in isopentane on dry ice or paraffin embedded. Free-floating 30 μm brain sections, slide-fixed 10 μm pituitary or PVN containing sections, and 8 μm paraffin WAT or BAT sections were used for histology and IHC. For IF and 3,3′-diaminobenzidine-based immunostainings, sections were treated as previously described [48] and probed with specific antibodies ( Supplementary Table 3 ). All fluorescent images were taken on LSM710 Meta confocal microscope (Carl Zeiss) mounting 40 × /0.75 NA and 63 × /1.4 NA plan-apochromat objectives (Carl Zeiss) or a Leica DM6000 with automated stage and then deconvoluted using the Leica Software. Bright field images were taken using an AxioScope microscope (Carl Zeiss) mounting 20 × /0.8 NA and 40 × /0.75 NA plan-apochromat objectives (Carl Zeiss), coupled with an AxioCam ICC1 colour camera (Carl Zeiss). Colocalization studies Serial coronal cryosections (10 μm) were collected on superfrost slides. Three sections spaced 80 μm apart and clearly containing the PVN were used for further analysis. Stained sections were imaged using a Zeiss LSM 710 confocal microscope, and double-labelled cells were counted in an area of 0.124 mm 2 per section in the dorso-medial AHN (defined by the region in between and ventrally to the PVN and the fornix). CCK-YFP fibre quantification Cryosections (10 μm) were collected on superfrost plus slides. Eight sections per mouse from each hemisphere spaced 60 μm apart and containing the PVN were stained for YFP, CRH and Neurotrace fluorescent Nissl (Invitrogen). Images of the PVN were taken on a Leica DM6000 with automated stage and deconvoluted using the Leica Software. The density of YFP positive fibres was analysed by ImageJ software. pERK immunostaining Cryosections (15 μm) were collected on superfrost plus slides. From each hemisphere, three sections spaced 120 μm apart and containing the PVN were used for each mouse. Sections were treated for 10 min in 100% methanol at −20 °C and then processed for diaminobenzidine staining with a pErk1/2 antibody (1:500 Cell Signaling #4370). Integrated staining density was quantified by ImageJ software. Cell counts The number of recombined (YFP-positive) and GR-positive neurons in the peri-PVN and AHN was determined in four mice per genotype (2–4-month-old male and female mice) using design-based stereology with the optical fractionator method. Serial coronal 10 μm cryosections were collected on superfrost slides through the whole PVN and AHN. After appropriate antibodies staining every third section was counted with an unbiased counting frame sized 40 × 40 μm with a grid size of 70 × 70 μm. The frames were randomly positioned using the ‘Unbiased counting frame’ macro in ImageJ (NIH). The dissector height was 6 μm with guard zones of 2 μm. Cells were counted in each frame according to the optical fractionator counting rules. The coefficient of error was calculated for each animal and did not exceed 0.07. The PVN and the third ventricle on the medial and rostral side, 550 μm lateral to the third ventricle and 700 μm ventral to the PVN-defined boundaries. The PVN was excluded from the analysis. Synaptic innervations The number of VGAT terminals on PVN CRH neurons was manually counted. CRH neurons were defined by CRH immunoreactivity and the whole cell body was defined by Neurotrace fluorescent Nissl staining. VGAT terminals touching CRH cell bodies were manually counted on 10 neurons per animal from 6–8 serial sections, 10 μm thick and spaced 60 μm apart, per animal ( n =4 for each genotype). Adrenal morphology Adrenals were dissected from perfused adult control and mutant mice (2-, 3- and 5-month-old male and female mice) and fixed overnight in 4% PFA/PBS, pH7.4. Adrenals were then dehydrated, paraffin-embedded and sectioned at 8 μm serial sections. Haematoxylin-Eosin staining was performed to visualize morphology. The thickness of the ZF was calculated using the measurement tool in either Image J ( http://imagej.nih.gov/ij/ ) or Photoshop, and it was defined as the mean of nine measurements across the middle of the gland per mouse (three sections per adrenal spaced 72 μm a part, three images per section covering the whole profile of the cortex). The measurements per adrenal were averaged, before values of both adrenals/mouse were averaged. Both genders showed significant adrenal hypertrophy in the Trkb Cck-KO mice. Liver morphology Tissue slabs of liver were dissected, fixed overnight in 4% PFA/PBS, pH7.4, cryoprotected in 30% sucrose and frozen in OCT. Cryosections of 10 μm were collected on superfrost slides and stained either with Haematoxylin/Eosin or Oil Red O/Haematoxylin. For the latter, sections were rinsed in distilled water, equilibrated briefly in propylene glycol and incubated for 3 min in 0.5% Oil Red O in propylene glycol at 60 °C. Slides were then washed in 85% propylene glycol and distilled water, haematoxylin stained and mounted with glycerine jelly. The Oil Red O signal was analysed with ImageJ software in five images obtained from different regions of the liver. A threshold in the YUV colour space identifying the Red Oil O signal was applied with the ‘Threshold Colour’ plugin as described [59] . Briefly, the U and V colour space was used to define the colour corresponding to the Oil Red O signal. The threshold for the signal intensity was set in the Y space that corresponds to the overall brightness. The total area covered by Oil Red O signal was determined with the particle analysis tool. To compare controls on vehicle to controls on drug values were normalized to the mean of the control vehicle group. To compare mutants on vehicle versus mutants on drug, both groups were normalized to the mean of their respective control group. In situ hybridization Brains from decapitated mice were freshly frozen. RNA in situ hybridization was performed on 10 μm cryosections (fixed for 15 min with ice-cold 4% PFA/PBS pH7.4) using digoxigenin-labelled (DIG-RNA labelling kit, Roche) antisense/sense probes for Trkb , Crh , Avp and Enkephalin . Probes were generated by PCR amplification from commercial or in-house subclones ( Supplementary Table 4 ). For the combined Trkb in-situ hybridization and GFP IF brains were processed as described for IHC, except 8 μm sections were placed onto superfrost plus slides (VWR). For Crh , Avp and Penk in-situ hybridizations, brains were not prefixed, but snap frozen in OCT for 25 s in isopentane on dry ice. Sections (10 μm) were fixed for 15 min in 4% PFA/PBS immediately prior to staining, washed in PBS and, only in the case of prefixed sections, treated with 10 μg ml −1 Proteinase K (Roche) in PBS for 6 min at 37 °C. Slides were fixed in 4% PFA for 10 min, washed with PBS and equilibrated for 5 min in 0.1 M triethanolamine pH 8.0, acetylated for 10 min in 0.25% acetic anhydride in 0.1 M triethanolamine pH 8.0, and washed in PBS. Sections were then prehybridized for 2 h at 58 °C in hybridization buffer (50% (vol/vol) formamide, 5 × SSC, 5 × Denhardt’s solution, 250 μg ml −1 tRNA, 100 μg ml −1 salmon sperm) in a humidified chamber (50% (vol/vol) formamide, 5 × SSC). Probes were diluted to 800 ng ml −1 in hybridization buffer, incubated for 5 min at 80 °C, chilled on ice prior to addition of probes (150 μl) and hybridized in a humidified chamber at 58 °C for 24–40 h. Post-hybridization washes consisted of 2 × SSC at room temperature (RT), 2 × SSC at 65 °C and 0.1 × SSC at 65 °C. Sections were then washed in PBS, blocked for 1 h in 10% (vol/vol) normal sheep serum (Millipore), 0.1% (vol/vol) Tween-20 in TBS, pH 7.5. Alkaline phosphatase-conjugated DIG antibody (Roche) (1:1,000 in blocking solution) was applied to the sections, which were incubated over night at 4 °C in a humidified chamber. Sections were washed in TBST (TBS, 0.1%(vol/vol) Tween-20, pH7.5), placed for 5 min in freshly prepared NTMT buffer (100 mM Tris-HCl pH 9.5, 100 mM NaCl, 100 mM MgCl 2 , 0.1% (vol/vol) Tween-20) and then in NTMT buffer with 5 mM levamisole (Sigma). For colour development, NTMT buffer containing 3.75 μl ml −1 BCIP, 5 μl ml −l NBT, 0.1% (vol/vol) Tween-20 and 5 mM levamisole was applied and sections incubated 2 h to overnight in a humidified chamber at RT until a signal was visible. Reactions were stopped by washing in 1 mM EDTA in PBS, followed by 95% (vol/vol) ethanol for several hours. Sections were then rinsed in PBS and mounted with Vectashield (Vector Laboratories). When IF was performed, the primary antibody was applied together with the anti-DIG antibody and the secondary antibody was applied for 2 h at RT, followed by washes in TBST before changing to NTMT buffer. Analysis of staining density and integrated density was performed using ImageJ. A threshold in the YUV colour space identifying the BCIP/NBT signal was applied using the ‘Threshold Colour’ plugin (see above). The stained area and density was then measured with the measurement tool including areas bigger than 25 μm 2 . Three sections containing the PVN and spaced 80 μm apart were analysed per mouse. PVN tissue punches and qRT–PCR analysis Both male and female animals at 5 months of age were culled by cervical dislocation and brains were quickly dissected and frozen. From each animal four 200 μm fresh-frozen coronal sections containing the PVN (bregma −0.18 to −1.155, Allen Mouse Brain Atlas) were collected on a cryostat CM3030 S (Leica Biosystems). Punches were isolated using Gilson CP-100 positive-displacement tips. Total RNA was isolated using Trizol (Invitrogen) and cDNA synthesis was achieved using Superscript VILO cDNA synthesis kit (Invitrogen) as per the manufacturer’s instructions. Quantitative PCR was performed using UPL assay (Roche) on the 7500 Fast Real Time PCR System (Applied Biosystems). All primers were designed using Universal ProbeLibrary Assay design Centre (Roche) ( Supplementary Table 4 ). Threshold cycle of C t value was set manually for each experiment and data was analysed using 7500 Fast Real Time PCR System software (System Biosciences). C t values of each gene were normalized to that of Tbp (Δ C t ) of a same sample. Data were arranged as fold difference between control and mutants by ΔΔ C t method. Food intake over several weeks Food intake was analysed in LabMaster metabolic cages (#995100-CA-T3, TSE Systems, Bad Homburg, Germany). Male mice at 2–3 and 7–8 months of age were housed individually and allowed to acclimatize in the chambers for at least 24 h with free access to food and water. Food intake on SC (#2018 global rodent diet, Teklad, 6% fat, 3.4 kcal g −1 ) was measured for 3 weeks. Two groups of mutants and controls were monitored in two independent experiments. The accumulated food intake corresponds to the total quantity of food consumed during the study period. Values were then normalized to the first week food intake of the control group to allow the two experiments to be combined. Mice were then transferred to a diet with 34% fat content (high-fat diet) (#TD.06414, Harlan Laboratories, Madison, USA, 5.1 kcal g −1 ) for 3 weeks. Food intake was averaged over the third week and compared with the average weekly food intake on a normal diet for each separate genotype. Circadian pattern of food intake was analysed on SC (2018 Teklad Global 3.4 kcal g −1 ). Food intake in the dark period (12 h, 19:15 to 07:15) and in the light period (12 h, 07:15 to 19:15) was measured over a week. Indirect calorimetry with food intake and home cage activity Metabolic rate, food intake and home cage activity measurements were performed simultaneously in 7.1 l chambers of the PhenoMaster open-circuit calorimetry (PhenoMaster System, TSE Systems). Mice were kept at 22–24 °C and were allowed to acclimatize in the chambers for at least 24 h. Food and water were provided ad libitum in the appropriate devices and measured by the build-in automated scales. The system was further equipped with an infrared light-beam frame to determine the home cage activity (ActiMot2, TSE Systems GmbH, Bad Homburg, Germany). Data were collected for at least 48 h. Parameters were normalized to FFM+0.2FM (FFM, FM obtained by NMR), as this has been suggested to best represent the metabolically active tissue mass [59] . Body composition analysis NMR was employed to determine whole-body composition of live animals using the NMR Analyzer minispec mq7.5 (Bruker Optik, Ettlingen, Germany). Glucose tolerance test For glucose tolerance tests, 3- and 9-month-old male mice were starved for 6 h at the beginning of the light phase. Animals were injected with glucose (2 g kg −1 body weight, 20% glucose; Delta Select) into the peritoneal cavity. Glucose levels were determined in blood collected from the tail tip immediately before, and 15, 30, 60 and 120 min after the injection using a hand-held glucose meter (Bayer Contour, Bayer Health Care, Leverkusen, Germany). Hormones and metabolites For morning CORT and ACTH serum measurements, 5-month-old male and female animals were quickly decapitated and trunk blood collected in 50 μl of 0.5 M EDTA and a proteinase inhibitor cocktail (Sigma). For all other measurements including insulin and leptin levels, animals were sacrificed by CO 2 and blood was collected by cardiac puncture into 1/10 volume of 0.5 M EDTA and a proteinase inhibitor cocktail (Sigma). Blood was separated by centrifugation for 10 min at 2,000 r.p.m., the serum frozen on dry ice and stored at −80 °C. Serum ACTH was determined by enzyme immunoassay (EIA) (Phoenix Pharmaceuticals) and RIA (Diasorin) according to manufacturer’s instructions. Serum CORT (Immunodiagnostic Systems) insulin and leptin (both Millipore) were determined by EIA. Serum glucose was analysed using the Glucose QuantiChrom Assay Kit (BioAssay Systems). Mifepristone treatment Old obese (9 M) male mutants and controls (3–6 per group) were treated for 8 weeks with either 10 mg kg −1 mifepristone (also known as RU-486) or vehicle administered via the drinking water to avoid stress through repeated handling. Drinking water was supplemented with 0.2% ethanol and adjusted to pH 3.5 to prevent the drug from precipitating; 0.2% ethanol pH 3.5 was used as vehicle. The drug dose, 10 mg kg −1 , was calculated on a daily water intake of 4 ml–a value determined using the metabolic cages. Body weight was measured once per week. Behavioural tests All animals (5-month-old male mice, or 2- and 8-month-old male mice for home cage activity) were habituated to the test room for 30 min prior to testing. OF test: animals were placed in the middle of the OF arena (50 × 50 × 22 cm) illuminated with 150–200 Lux and allowed to freely explore for 30 min. Animals were tracked using the TSE VideoMot2 system and light-beam frames placed around the arena measured rearing. Time spent in the border and centre of the OF, number of visits to the centre, total distance travelled and rearing was automatically calculated using the TSE VideoMot2 software. Elevated plus maze test: animals were placed in the centre of the maze and tracked for 5 min using the TSE VideoMot2 system. Time spent in each arm or the centre and visits to each arm were calculated using the TSE VideoMot2 software. Acute restraint stress: 4-month-old female mice were restrained for 20 min in a restrainer and immediately sacrificed afterwards by CO 2 . Blood was collected by cardiac puncture; serum was processed for ACTH and CORT measurements as described above. Statistical analysis We performed statistical analysis by using Statview software. Two-way ANOVA using genotype, and either diet or drug treatment, as independent variables was used for data analysis of body weight and analysis of lipogenesis by WBs. Where significant effects were found, a post-hoc Fisher’s PLSD or Student’s t -test was performed and P -values and degrees of freedom reported. ANCOVA was used for testing interaction of lean body mass and genotype on EE. Body weight and body composition data, food intake, weight gain, hormone and glucose levels, adrenal morphology, tissue weights, in-situ staining density, qRT–PCR, stereology data, synaptic density, WBs quantifications, Oil-Red-O content, locomotor activity and behavioural parameters were analysed by two-tailed unpaired Student’s t -test. Data are presented as mean±s.e.m. or s.d. as specified in figure legends. The variance between groups was tested using Bartlett’s test in Statview and was confirmed in all data sets used in this study. P <0.05 was considered to be statistically significant. We did not use statistical methods to predetermine sample size. Sample sizes were based on pilot experiments and previous studies of similar nature [60] . We did not use randomization in this study, but for each experiment all genotypes were represented. Investigators were blind to genotype in all experiments, samples/slides were labelled with numbers not genotype and results were only allocated to genotypes after completing the analysis. Normal distribution was verified by using the Kolmogorov–Smirnov normality test in Statview. How to cite this article: Geibel, M. et al. Ablation of TrkB signalling in CCK neurons results in hypercortisolism and obesity. Nat. Commun. 5:3427 doi: 10.1038/ncomms4427 (2014).